Mapping the spatial distribution of charge carriers in quantum-confined heterostructures Quantum-confined nanostructures are considered ‘artificial atoms’ because the wavefunctions of their charge carriers resemble those of atomic orbitals. For multiple-domain heterostructures, however, carrier wavefunctions are more complex and still not well understood. We have prepared a unique series of cation-exchanged Hg x Cd 1− x Te quantum dots (QDs) and seven epitaxial core–shell QDs and measured their first and second exciton peak oscillator strengths as a function of size and chemical composition. A major finding is that carrier locations can be quantitatively mapped and visualized during shell growth or cation exchange simply using absorption transition strengths. These results reveal that a broad range of quantum heterostructures with different internal structures and band alignments exhibit distinct carrier localization patterns that can be used to further improve the performance of optoelectronic devices and enhance the brightness of QD probes for bioimaging. Semiconductor quantum dots (QDs) have recently attracted broad attention for applications in bioimaging, light-emitting devices, photovoltaics and quantum computing [1] , [2] , [3] , [4] , [5] , [6] , [7] , [8] , [9] , [10] . Compared with bulk semiconductor crystals, these nanocrystals exhibit unique optical and electronic properties, including size-tunable bandgaps and fluorescence emission, ultrafast charge-transfer rates and decreased lasing thresholds [9] , [10] , [11] , [12] , [13] , [14] , [15] , [16] , [17] . These properties largely arise from the quantum confinement effect, in which electronic charge carriers (electrons and holes) are spatially confined because of the small crystal size, similar to a spherical ‘particle in a box.’ This confinement results in quantized electronic energy levels that are analogous to discrete electronic transitions of atoms in the gas phase. However, this analogy becomes much more complex for quantum-confined heterostructures containing multiple chemical or structural domains. In these composite nanomaterials, separate regions have distinct potential energies that shape the spatial distribution and transport behaviour of different charge carriers. For example, in core–shell heterostructures with a ‘type-I’ band alignment, the potential energy of the electron and hole is lowest in the same domain (for example, the core) and thus the electron and hole are colocalized, resulting in a high probability of radiative recombination and a fluorescence quantum efficiency that can approach unity [18] , [19] , [20] . In contrast, in core–shell heterostructures with ‘type-II’ band alignments, the potential energy minima for the electron and hole are in different domains, resulting in charge carrier separation, longer excited state lifetimes and broad wavelength tunability [21] . It is thus critically important to determine and control the spatial distribution patterns of charge carriers; however, at present there are few experimental approaches available for such fundamental studies. Scanning tunnelling microscopy with spectroscopy has been used to image specific wavefunctions but the technique is very challenging and has low throughput [22] . Computational modelling studies also provide insight; however, alone they are of only limited utility as continuum models do not account for microscopic structural attributes and immense computational power is needed to account for atomistic effects when large numbers of atoms are involved [23] . Here we report a simple semiempirical method based on quantum mechanical models of the effective mass approximation (EMA) and steady-state optical absorption measurements for mapping the wavefunctions of charge carriers in quantum-confined heterostructures. Specifically, we have prepared a unique series of cation-exchanged Hg x Cd 1− x Te heterostructures, for which quantum mechanical calculations are simplified and the electronic transition probabilities are solely dependent on the electron–hole overlap integral. For this series of heterostructures, we have experimentally measured the 1st and 2nd exciton transition intensities (oscillator strengths) as a function of both particle size and chemical composition. The results show that the oscillator strength of the 1st exciton peak is dependent on the relative electron–hole overlap, while the intensity of second exciton peak measures the absolute spatial localizations of the electron and hole. We have further carried out extensive work, both experimental and theoretical, on seven common core/shell heterostructures, demonstrating that the relationship between electronic transition strengths and charge-carrier distributions is generalizable to a broad range of core–shell and alloyed nanostructures. These fundamental insights are critical for patterning the shapes and spatial locations of charge carrier wavefunctions and for funneling oscillator strength into specific optical transitions, which will help to exploit the novel properties of quantum nanostructures for future use in optoelectronic devices, quantum computing, solar energy conversion as well as bioimaging. Wavefunction modelling In a single-electron hydrogenic atom (for example, H, He + , Li 2+ ) in the gas phase, the electron energy levels are quantized, leading to a discrete set of electronic orbitals (s, p, d, and so on) with distinct absorption transitions. In semiconductor QDs, the crystalline lattice of atoms provides a potential energy well for excited-state charge carriers (electrons and holes), which have analogous wavefunction shapes. 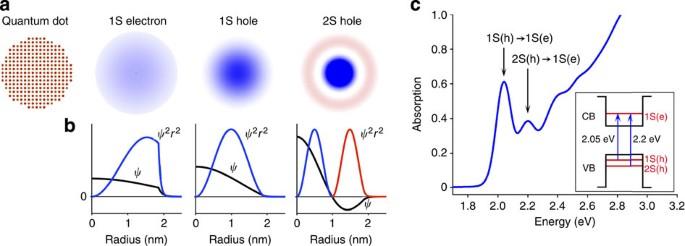Figure 1: Quantum mechanical modelling of charge carriers in quantum dot artificial atoms. (a) Cross-sectional views of a 3.8-nm CdTe quantum dot and its 1S(e), 1S(h) and 2S(h) wavefunctions; (b) corresponding wavefunction () and radial distribution function () plots; and (c) steady-state absorption spectrum showing the 1st exciton 1S(h)→1S(e) and the 2nd exciton 2S(h)→1S(e) transitions. The energy band diagram in the inset depicts these absorption transitions between quantum-confined electron (e) and hole (h) energy states. Black lines indicate potential energy wells in the CB and VB. For clarity, energy levels are not drawn to scale and higher energy levels are omitted. Figure 1a depicts the lowest-energy electronic energy states for the electron (1S) and hole (1S) in addition to the next highest energy state of the hole (2S) in a pure cadmium telluride (CdTe) QD; the shapes resemble the corresponding 1s and 2s atomic orbitals. Figure 1b depicts plots of the wavefunctions ( ) and radial distribution functions (RDF, ) of these carriers based on the EMA [24] . The 1S electron exhibits greater spatial confinement than the 1S hole because the effective mass of an electron ( m e =0.090) is much smaller than that of a hole ( m HH , heavy-hole effective mass is equal to 0.83; see Supplementary Table 1 ). As a result, the 1S electron density is distributed further away from the QD centre than the 1S hole state (see RDF plots). Figure 1: Quantum mechanical modelling of charge carriers in quantum dot artificial atoms. ( a ) Cross-sectional views of a 3.8-nm CdTe quantum dot and its 1S(e), 1S(h) and 2S(h) wavefunctions; ( b ) corresponding wavefunction ( ) and radial distribution function ( ) plots; and ( c ) steady-state absorption spectrum showing the 1st exciton 1S(h)→1S(e) and the 2nd exciton 2S(h)→1S(e) transitions. The energy band diagram in the inset depicts these absorption transitions between quantum-confined electron (e) and hole (h) energy states. Black lines indicate potential energy wells in the CB and VB. For clarity, energy levels are not drawn to scale and higher energy levels are omitted. Full size image Figure 1c shows a typical electronic absorption spectrum for a QD composed of II–VI materials (here CdTe), showing multiple distinct electronic transitions. Through comparisons with quantum mechanical models, the absorption peaks have been assigned to transitions between specific electronic energy levels ( Supplementary Fig. 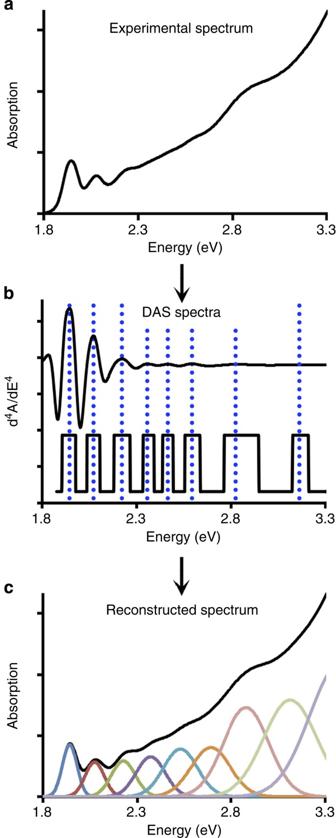Figure 2: Mathematical extraction of electronic transition energies and oscillator strengths for quantum-confined nanostructures. (a) An experimental spectrum is first subject to mathematical line narrowing through differentiation with respect to energy, resulting in differential absorption spectra. (b) Fourth derivatives are shown: the top is the original differential spectrum and the lower spectrum has been flattened to reveal lower intensity features. Vertical dotted lines indicate observed transition energies. (c) Using these energies, least squares fitting is used to reconstruct the original spectrum from a sum of Gaussian peaks with initial guesses for transition energies derived from differential absorption spectroscopy analysis. Integrated peak areas correspond to oscillator strengths. 1 and Supplementary Table 2 ). The 1st transition, 1S(h)→1S(e), arises from light absorption by an electron in the highest energy valence band (VB) state to transition to the lowest energy conduction band (CB) state [25] , [26] . This transition is also known as the 1st exciton peak, as it results in a bound electron–hole pair, a ground-state exciton. In the resulting 1S(e)1S(h) exciton, both carriers occupy 1S wavefunctions that substantially overlap in space. The 2nd exciton peak, 2S(h)→1S(e), arises from the excitation of an electron in the next highest VB level, again to the lowest energy CB level [27] , [28] . This results in a 1S(e)2S(h) exciton in which the hole occupies a 2S wavefunction. Both the 1S(h) and 2S(h) wavefunctions are spherically symmetric; however, the 2S(h) has a spherical nodal surface with zero electronic density separating regions of opposite polarity, as indicated by red and blue colours in Fig. 1a,b . Therefore, whereas the 1S(e)1S(h) exciton has strong electron–hole overlap, the 1S(e)2S(h) exciton overlap is small because of contributions from both constructive and destructive interference between the 1S electron and the two domains of opposite polarity of the 2S hole. As discussed below, the first and second exciton wavefunctions are greatly influenced by the nanocrystal structure and composition, and together can be used to map the spatial distributions of charge carriers in quantum nanostructures. Electronic transitions and oscillator strengths We are interested in measuring the oscillator strengths of the first and second excitonic transitions. Figure 2 depicts the two-step process to extract these values from QD electronic absorption spectra. The first step is to determine the electronic transition energies from often broad or apparently featureless absorption spectra, and then reconstruct the spectrum from a sum of Gaussian peaks, with integrated areas corresponding to transition oscillator strengths. Transition energy extraction is limited by spectral overlap between adjacent peaks. Peak width is a function of sample homogeneity (size, shape and composition), transition energy and homogeneous broadening effects. As a result, significant peak overlap is observed even for QD samples that are considered structurally homogeneous by current standards. Moreover, even if the spectral peaks are distinct, their maxima do not necessarily correspond with the true peak energy because contributing shoulders from neighbouring peaks can shift the observed peak centroid. To overcome this problem, we have used differential absorption spectroscopy (DAS) for mathematical narrowing of convolved peaks: even order derivatives (for example, 2nd, 4th derivatives) have substantially narrower peak profiles than those of the zeroth-order spectra (see Supplementary Methods for more details). Figure 2: Mathematical extraction of electronic transition energies and oscillator strengths for quantum-confined nanostructures. ( a ) An experimental spectrum is first subject to mathematical line narrowing through differentiation with respect to energy, resulting in differential absorption spectra. ( b ) Fourth derivatives are shown: the top is the original differential spectrum and the lower spectrum has been flattened to reveal lower intensity features. Vertical dotted lines indicate observed transition energies. ( c ) Using these energies, least squares fitting is used to reconstruct the original spectrum from a sum of Gaussian peaks with initial guesses for transition energies derived from differential absorption spectroscopy analysis. Integrated peak areas correspond to oscillator strengths. Full size image On the basis of analyses of synthetic spectra of QDs with known Gaussian transition energies, we have determined the spectral parameters for which transition energy and oscillator strength can be accurately measured. 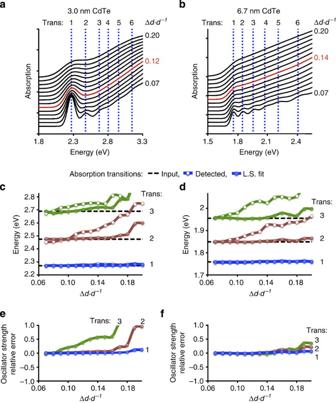Figure 3: Effect of quantum dot size dispersion on the extraction accuracy of electronic transition energies and oscillator strengths Spectra were generated from sums of Gaussian curves with contributing noise and widened according to specific dispersions of diameter (Δd·d−1).a,bshow the spectra that were generated from Gaussian peaks with energies noted by vertical dotted lines (transitions 1–6).c,dshow peaks that were extracted from the 4th derivatives of these spectra (coloured lines with open circles), and then fit to the original spectrum (coloured lines with closed circles), in addition to the input energy for each peak (dotted black lines).e,fdepict the relative oscillator strengths of the 1st (blue), 2nd (red) and 3rd (green) absorption transitions with size dispersion. Figure 3a,b shows synthetic spectra of two sizes of CdTe nanocrystals with a range of size dispersions, with vertical lines indicating input transition energies, numbered 1–6. We extracted the transition energies using the 4th derivative: Fig. 3c,d shows that the first exciton energy (blue curves) is at least 99% accurate (within 20–30 meV depending on size) even when the size dispersion is as large as 20% relative s.d. in diameter (Δ d·d −1 ) . The determined energy of the second exciton transitions using DAS is at least 99% accurate for Δ d·d −1 <11% (red curves, open circle markers). Spectral reconstruction through least squares fitting further improves the transition energy accuracy. Thus, we find that it is not necessary to determine the peak energy with very high accuracy but rather it is more important to determine the accurate number of peaks within a specific spectral window (see Supplementary Discussion ). The extracted energy provides an ‘initial guess’ for the energy; by allowing the energies to shift, the curve-fitting algorithm finds the original peaks. We show that even when the extracted 4th derivative is inaccurate by 90 meV, the fitting algorithm finds the original peak, within several meV (compare the open and closed circle markers in Fig. 3c,d ), and the resulting energies are at least 99% accurate for Δ d·d −1 ≤15%. We have also investigated whether experimental band narrowing through photoluminescence excitation (PLE) spectroscopy, rather than through DAS, could improve the resolution of contributing absorption peaks. As shown in Supplementary Fig. 2 , the low energy peaks were similar to those of the DAS spectra; this is consistent with previous PLE spectral analysis of CdTe nanocrystals by Zhong et al. [29] , as well as with theoretical predictions by Efros et al. [27] (see Supplementary Fig. 1 ). Figure 3: Effect of quantum dot size dispersion on the extraction accuracy of electronic transition energies and oscillator strengths Spectra were generated from sums of Gaussian curves with contributing noise and widened according to specific dispersions of diameter (Δ d·d − 1 ). a , b show the spectra that were generated from Gaussian peaks with energies noted by vertical dotted lines (transitions 1–6). c , d show peaks that were extracted from the 4th derivatives of these spectra (coloured lines with open circles), and then fit to the original spectrum (coloured lines with closed circles), in addition to the input energy for each peak (dotted black lines). e , f depict the relative oscillator strengths of the 1st (blue), 2nd (red) and 3rd (green) absorption transitions with size dispersion. Full size image Figure 3e,f depicts the error in calculated oscillator strength of the first three transitions of these nanocrystals, determined through least squares fitting. At low size dispersions, all spectra are accurately fit, but deviations arise with increasing size dispersion. Higher accuracy is obtained for larger nanocrystals compared with smaller nanocrystals with the same size dispersion, as peaks are less ‘hidden’ by the first exciton for larger sizes. The 1st and 2nd exciton oscillator strengths are found to be accurate (within 5% of the input value) for 3.0-nm nanocrystals with Δ d·d −1 ≤12% and for 6.7-nm nanocrystals with Δ d·d −1 <14%. The corresponding spectra are marked in red in Fig. 3a,b . It is surprising that even for these somewhat featureless spectra, the subtle changes in curvature provide sufficient information about the underlying peaks, which allow us to determine the number and strength of peaks. All QDs analysed in this paper have spectral bandwidths narrower than these threshold values, such that their transition energies and oscillator strengths are determined with ≥99% and ≥95% accuracy, respectively. Core–shell and alloyed heterostructures To understand how the shapes of potential energy wells in complex heterostructures dictate carrier wavefunction shapes and oscillator strengths, we have carried out systematic experimental and theoretical studies of core–shell and cation-exchanged QDs. We first discuss cation-exchanged Hg x Cd 1−x Te heterostructures as a model system because they are nearly free from lattice strain and quantum mechanical calculations are simplified. For colloidal synthesis we start with monodisperse CdTe nanocrystals with tunable size and exchange Cd 2+ ions in the lattice with Hg 2+ ions as previously reported [30] . Energy-dispersive X-ray spectroscopy (EDX) and inductively coupled plasma mass spectrometry (ICP-MS) demonstrate the substitution of cadmium for mercury ( Supplementary Figs 3 and 4 ). Cubic CdTe and HgTe are fully miscible as a ternary alloy and have nearly identical lattice constants ( a CdTe =6.48 Å, a HgTe =6.46 Å); therefore, the bond lengths and crystallinity do not substantially change with mercury exchange, as verified by powder X-ray diffraction ( Supplementary Fig. 5 ) and transmission electron microscopy ( Supplementary Figs 6 and 7 ). Large CdTe nanocrystals form core–shell structures, as determined by Raman scattering ( Supplementary Fig. 8 ): the CdTe phonon modes remain after substantial cation exchange but are broadened because of reduced domain size, and new broad scattering modes arise corresponding to those of HgTe. Furthermore, a kinetic analysis of exchange reactions reveals that for larger nanocrystals (>5 nm), exchange occurs rapidly (minutes) until a monolayer has been formed, after which the exchange rate is substantially reduced ( Supplementary Fig. 9 ). This is not the case for smaller nanocrystals, for which exchange beyond a monolayer is rapid; these particles have a dynamic structure with significantly higher ion mobility that leads to homogeneous alloying, as described below. Cation exchange leads to significant alterations to the optical spectra because of the very different bandgap energies and electron–hole masses of CdTe and HgTe. These changes depend on whether the final structure is a core–shell or alloy ( Fig. 4a ). The bulk bandgap energy of CdTe is 1.5 eV, whereas that of HgTe is −0.15 eV (a near-zero bandgap in which the bottom of the CB is almost aligned with the top of the VB). Thus, as shown in Fig. 4b (energy band structures based on EMA calculations), cation substitution of Cd 2+ by Hg 2+ in CdTe nanocrystals leads to a decrease in bandgap energy and altered degree of carrier confinement. For homogeneous alloys, the CB shifts to lower energy and the VB shifts to higher energy. This is not the case for the core–shell products, for which two separate domains emerge: the electron now has a lower energy level in the shell region that results in a substantial reduction in bandgap energy. Although the hole well is also deepened, the 1S and 2S hole levels do not significantly change in energy relative to the CdTe nanocrystals or redistribute to the shell because the small effective mass of the hole in HgTe ( m HH =0.03) offsets changes in potential well depth. Thus, the electron is redistributed to the shell region, whereas hole states remain distributed throughout the nanocrystal, resulting in a pseudo-type II band alignment with a spatially indirect bandgap. 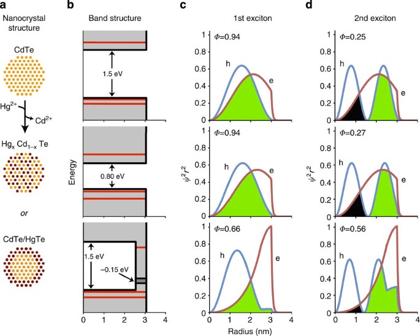Figure 4: Structure and charge carrier properties of CdTe QDs and cation-exchanged HgxCd1−xTe QDs. (a) Schematic illustrations of CdTe QDs, homogeneous alloy HgxCd1−xTe QDs, or core–shell CdTe/HgTe QDs generated through Cd2+replacement by Hg2+. (b) Energy band diagrams showing the valence and conduction bands (grey), potential energy wells (black lines) and quantum-confined kinetic energy levels (red lines) of electrons and holes in each QD, as calculated using the effective mass approximation. (c,d) RDF (, nm−1) plots of the electron (e) and hole (h) for the 1st and 2nd excitons. Wavefunction overlap integrals (φ) are also provided. Constructive overlap is schematically depicted as green and destructive overlap is black. Figure 4: Structure and charge carrier properties of CdTe QDs and cation-exchanged Hg x Cd 1−x Te QDs. ( a ) Schematic illustrations of CdTe QDs, homogeneous alloy Hg x Cd 1− x Te QDs, or core–shell CdTe/HgTe QDs generated through Cd 2+ replacement by Hg 2+ . ( b ) Energy band diagrams showing the valence and conduction bands (grey), potential energy wells (black lines) and quantum-confined kinetic energy levels (red lines) of electrons and holes in each QD, as calculated using the effective mass approximation. ( c , d ) RDF ( , nm − 1 ) plots of the electron (e) and hole (h) for the 1st and 2nd excitons. Wavefunction overlap integrals (φ) are also provided. Constructive overlap is schematically depicted as green and destructive overlap is black. Full size image The EMA predicts that the potential energy shapes for the two possible products will yield substantial differences in carrier wavefunction shapes for the 1st and 2nd excitons ( Fig. 4c,d ) that will lead to alterations in exciton overlaps that can be directly measured by changes in absorption oscillator strength. For core CdTe nanocrystals, the 1S(e) and 1S(h) states of the 1st exciton initially strongly overlap (overlap integral Φ 1 =0.94, Fig. 4c ), whereas for the 2nd exciton, 1S(e) overlaps both with regions of negative and positive polarity of 2S(h), yielding a small net overlap ( Φ 2 =0.25, Fig. 4d ). If the resulting Hg x Cd 1−x Te nanocrystal is a homogeneous alloy, the overlaps do not substantially change compared with the CdTe nanocrystal ( Φ 1 =0.94, Φ 2 =0.27). However, for the core–shell CdTe/HgTe nanocrystals, the electron migrates to the shell region and the hole remains distributed throughout the nanocrystal so the 1st exciton overlap decreases (to Φ 1 =0.66) and the 2nd exciton overlap increases (to Φ 2 =0.56) because the electron moves away from the 2S hole node to increase overlap with a region of like polarity and reduce overlap with regions of opposite polarity. Thus, for cation-exchanged core–shell nanostructures, the 1st exciton transition strength is predicted to decrease and the 2nd exciton strength will increase (more than twofold); these will not substantially change for an alloyed structure. This decrease in oscillator strength of the 1st exciton peak has been widely reported for type-II heterostructures [21] , [31] , [32] . However, the 2nd exciton peak has not been explored in this context but should be a more specific and sensitive ‘reporter’ for localization because of the capacity to either decrease or increase depending on small shifts in wavefunction distribution. Whereas the 1st exciton peak oscillator strength can reveal a relative change in electron–hole overlap, changes in the 2nd exciton peak provide a sensitive probe for the absolute spatial localization of the electron or hole in the core or shell. We compared predictions from the EMA model with experimental data from CdTe→Hg x Cd 1−x Te cation-exchanged nanocrystals. 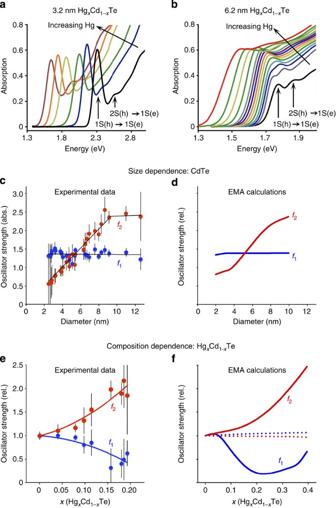Figure 5: Optical absorption spectra during HgxCd1−xTe cation exchange. Mercury cation exchange was performed on CdTe cores with a diameter of (a) 3.2 nm or (b) 6.2 nm. For 3.2-nm nanocrystals, absorption increases substantially at high energy with little change in band-edge oscillator strength. For the 6.2-nm nanocrystals, the 2nd exciton peak becomes dominant with increasing mercury content. (c) Experimental oscillator strengths of the 1st exciton transition (f1, blue) and 2nd exciton transition (f2, red) for CdTe QDs with sizes from ~2 to 12 nm diameter, in absolute units. (d) Theoretical EMA calculations (plotted in relative units). (e) Experimental oscillator strengths of the 1st and 2nd exciton transitions for large CdTe nanocrystals (6.2 nm) after cation exchange. (f) Theoretical EMA calculations (plotted in relative units). For plots inc–f, solid curves show values for core–shell nanocrystals and dotted lines indicate values for homogeneous alloys. Error bars are s.d. Figure 5a shows that mercury exchange of 3.2-nm CdTe QDs leads to a monotonic shift of the absorption spectra to lower energies, and the major excitonic transitions remain discrete and with similar intensities and bandwidths (the molar QD concentration is identical for all spectra plotted on the same chart herein), indicating uniform cation exchange across the nanocrystal ensemble. Different trends were observed when the same experiment was performed on larger nanocrystals (6.2 nm, Fig. 5b ): the 1st exciton transition initially exhibited little change in energy while absorption at higher energies increased. In addition, the 2nd exciton peak increased in intensity and merged with the 1st exciton peak. This trend was similar for 8.4-nm nanocrystals ( Supplementary Fig. 10 ). Figure 5: Optical absorption spectra during Hg x Cd 1−x Te cation exchange. Mercury cation exchange was performed on CdTe cores with a diameter of ( a ) 3.2 nm or ( b ) 6.2 nm. For 3.2-nm nanocrystals, absorption increases substantially at high energy with little change in band-edge oscillator strength. For the 6.2-nm nanocrystals, the 2nd exciton peak becomes dominant with increasing mercury content. ( c ) Experimental oscillator strengths of the 1st exciton transition ( f 1 , blue) and 2nd exciton transition ( f 2 , red) for CdTe QDs with sizes from ~2 to 12 nm diameter, in absolute units. ( d ) Theoretical EMA calculations (plotted in relative units). ( e ) Experimental oscillator strengths of the 1st and 2nd exciton transitions for large CdTe nanocrystals (6.2 nm) after cation exchange. ( f ) Theoretical EMA calculations (plotted in relative units). For plots in c – f , solid curves show values for core–shell nanocrystals and dotted lines indicate values for homogeneous alloys. Error bars are s.d. Full size image We extracted absorption transition energies and transition oscillator strengths for these Hg x Cd 1−x Te QDs, monitoring each specific transition that was originally assigned in CdTe as we incrementally increased mercury content, traced by elemental analysis (see Supplementary Fig. 4 ). For small nanocrystals (<5 nm), all of the CdTe core transitions shifted to lower energies nearly linearly with increasing Hg content ( Supplementary Fig. 11a ). This is expected for homogeneous alloys with similar VB structures, that is, common-anion alloys (the VB predominantly arises from the anion p orbitals). In contrast, larger nanocrystals exhibited nonlinear transition trends with increasing Hg content, with several peaks becoming too closely spaced in energy to be distinguished ( Supplementary Fig. 11b ). To reconstruct the band edges for oscillator strength calculation, at least four peaks were used for small nanocrystals and at least seven peaks were used for large nanocrystals (see Supplementary Methods ) and the oscillator strengths of the 1st and 2nd exciton transitions ( f 1 and f 2 , respectively) were calculated from the integrated peak areas [33] . Figure 5c shows oscillator strengths per QD for pure CdTe nanocrystals ( x =0, no mercury) with diameters between 2 and 12 nm. The oscillator strength of the 1st exciton transition is nearly constant with size ( f 1 =1.33±0.10), as predicted by the EMA ( Fig. 4b ). These values are in close agreement with those found previously for CdTe nanocrystals [34] , and follow trends previously observed for CdS [35] and InAs [36] . Unlike f 1 , f 2 is almost linearly proportional to diameter ( f 2 =0.239 d nm − 1 ) for sizes smaller than 9 nm. The increasing value of f 2 relative to f 1 with diameter is apparent when comparing the spectra of 3.2 and 6.2 nm CdTe nanocrystals in Fig. 5a,b . A trend of increasing f 2 with size was previously reported for CdSe nanocrystals by Klimov [33] ; however, we are not aware of other experimental investigations of f 2 for colloidal QDs. A two-band interacting EMA model for these transition oscillator strengths shows a similar trend in Fig. 5d . The disproportionate concentration of oscillator strength in the 1S(h)→1S(e) transition for small nanocrystals compared with the 2S(h)→1S(e) and higher energy transitions is a result of the near-independence of the 1st exciton overlap with QD size. This is in contrast to the 2nd exciton, for which small changes in electron or hole confinement lead to substantial changes in net overlap because of the presence of the 2S hole node. It is notable that the experimental trend in the 2nd exciton oscillator strength could not be reproduced in EMA models unless band interactions were taken into account. The resulting wavefunctions showed that interactions become important for larger sizes, as the relatively unconfined 2S hole attracts the 1S electron closer to the centre of the nanocrystal as the node spreads farther from the centre, increasing net overlap with increasing size. We note that the CdTe nanocrystals used in this work are slightly prolate (with an aspect ratio of ~1.3). This would result in anisotropic wavefunctions for which one dimension is elongated relatively to the other two dimensions. However, Norris et al. [37] have shown that for nonspherical CdSe nanocrystals (also with an aspect ratio near 1.3), the transition energy and peak splitting are largely unaffected by this degree of anisotropy. For nonsperical CdTe, EMA calculations show a roughly fivefold smaller splitting energy compared with that of prolate CdSe [38] . This result is consistent with our data, in that we observed no spectral peak splitting or transition energy shifts in comparison with predictions from theory and previous PLE spectroscopic results ( Supplementary Fig. 1 ) [27] , [29] . For the Hg x Cd 1− x Te cation-exchanged QDs, trends in f 1 and f 2 with mercury content were strongly dependent on nanocrystal size and the cation exchange rate. We investigated three cation exchange methods: (1) in water using mercury–thioglycerol complexes, (2) in nonpolar solvents using mercury octanethiolate and (3) in nonpolar solvents using highly reactive mercury acetate. Methods 1 and 2 allowed slow, controlled exchange yielding spectral shifts over hours to days, whereas method 3 resulted in a rapid spectral red-shift in just seconds; we designate these two exchange regimes ‘slow’ or ‘fast.’ For large nanocrystals, the result of fast and slow exchange was similar: f 1 decreased and f 2 increased with increasing mercury content ( Fig. 5e ). This trend was anticipated for core–shell nanocrystals: in Fig. 5f , solid lines depict EMA predictions for core–shell nanocrystals and dotted lines show homogeneous alloys, which change very little with increasing mercury content. For small nanocrystals, slow and fast exchange modes were markedly different. For slow exchange, f 1 and f 2 only changed slightly with increasing mercury content ( Supplementary Fig. 12 ), in accord with the formation of a homogeneous alloy, whereas for fast exchange, f 1 decreased and f 2 increased, reflecting a core–shell structure. For fast exchange, f 1 and f 2 slowly approached their original values, suggesting redistribution of mercury to the core and suggesting that the cation exchange process is kinetically controlled by a balance between surface exchange and diffusion/alloying within the nanocrystal, which is consistent with our kinetic exchange experiments ( Supplementary Fig. 9 ). Diagrams of charge carrier localization We next determined how oscillator strength analyses could be used as a generalizable tool for a wide variety of core–shell QDs. Validation with cation-exchanged Hg x Cd 1− x Te was a critical step because the photophysics of this system are simple: the total number of oscillators (that is, atoms or bonding electrons) and the size does not change, and thus f is solely dependent on the electron–hole overlap integral. In addition, this system is nearly free from lattice strain because CdTe and HgTe have similar cubic lattice constants. This is important because strain is expected to strongly impact the optical and electronic properties of lattice-mismatched core–shell systems because of alterations to bond lengths that shift electronic energy bands, warp bands at interfaces and split degenerate hole states [11] , [32] . Typically, core–shell materials are grown through epitaxial deposition of a shell on a preformed core, such that the total number of oscillators and the nanocrystal size change, and strain effects are often dramatic when using lattice-mismatched materials [11] , [31] . To examine these effects with respect to f 1 and f 2 , we prepared seven core–shell nanocrystals starting from highly homogeneous cores: CdTe/CdSe, CdSe/CdS, CdSe/ZnTe, CdSe/ZnS, CdS/CdSe, CdS/ZnSe and CdS/ZnS. Similar to CdTe, the 1st and 2nd exciton transitions of CdS and CdSe were previously assigned as the 1S(h)→1S(e) and 2S(h)→1S(e) transitions, respectively. So that we did not have to calculate absolute oscillator strengths, we simply calculated relative oscillator strengths (ROSs) per QD, defined as: f rel was calculated from concentration-normalized absorption spectra obtained during shell growth. Spectra were reconstructed through least-squares fitting of a sum of Gaussian curves to determine and . As shown in Fig. 6 , trends were clear for specific electron–hole localization regimes with just 0–1.2 ML of shell growth, and match expected oscillator strength relationships based on the EMA model. Homoepitaxy (simply growing CdTe on CdTe cores, Fig. 6a,e ) did not alter but resulted in a monotonic increase in , in accord with Fig. 5c,d . Type I QDs with strong localization of the electron and hole in the core showed little change in and with increasing shell thickness (CdSe/ZnS, panels b,f). Type II h/e QDs with core-localized hole and shell-localized electron showed a strong decrease in and a strong increase in with increasing shell thickness (CdTe/CdSe, panels c,g), much like CdTe/HgTe nanocrystals with large cores. Type II e/h QDs with core-localized electron and shell-localized hole showed little change in and a strong decrease in with increasing shell thickness (CdSe/ZnTe, panels d,h) as the 2S hole migrates towards the shell, increasing overlap between the electron wavefunction maximum and the hole node. We also investigated type I core/shell QDs for which both the electron and hole localize to the shell, often called quantum wells (CdS/CdSe, Supplementary Fig. 13d,h ). 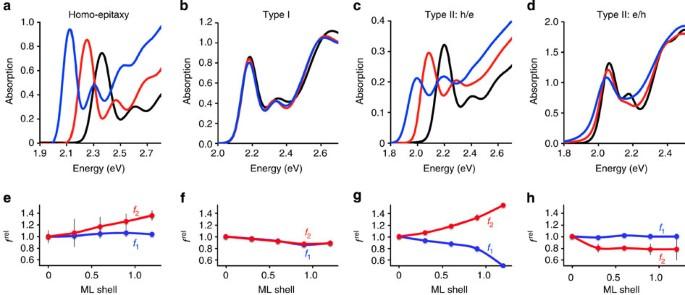Figure 6: Epitaxial shell growth in four different carrier localization regimes. Absorption spectra are shown ina–dand relative oscillator strengths are plotted for the 1st exciton transition () and 2nd exciton transition () ine–g. Regimes are designated as: (a,e) homoepitaxial growth (CdTe/CdTe), (b,f) Type I with electron and hole in the core (CdSe/ZnS), (c,g) Type II h/e with the hole in the core and electron in shell (CdTe/CdSe) and (d,h) Type II e/h with the electron in the core and hole in the shell (CdSe/ZnTe). Absorption spectra show cores with nominal shell thicknesses of 0 (black), 0.6 (red) and 1.2 (blue) monolayers (ML). Error bars are s.d. Figure 6: Epitaxial shell growth in four different carrier localization regimes. Absorption spectra are shown in a – d and relative oscillator strengths are plotted for the 1st exciton transition ( ) and 2nd exciton transition ( ) in e – g . Regimes are designated as: ( a , e ) homoepitaxial growth (CdTe/CdTe), ( b , f ) Type I with electron and hole in the core (CdSe/ZnS), ( c , g ) Type II h/e with the hole in the core and electron in shell (CdTe/CdSe) and ( d , h ) Type II e/h with the electron in the core and hole in the shell (CdSe/ZnTe). Absorption spectra show cores with nominal shell thicknesses of 0 (black), 0.6 (red) and 1.2 (blue) monolayers (ML). Error bars are s.d. Full size image These trends are best summarized on a ROS chart of versus ( Fig. 7 ), which graphically depicts localization regimes based on capping-induced redistribution of oscillator strength. A capping experiment starts with ‘origin’ coordinates of (1,1) for the core nanocrystal, and shell growth results in a trajectory moving away from this initial point along a specific path of carrier localization regimes. These plots clearly distinguish between the two type II regimes (e/h versus h/e), which is not possible solely through an examination of the 1st exciton peak, and distinguishes the two type I regimes for which the carriers are localized in the core (eh/o) or in the shell (o/eh). The magnitude of localization is also depicted; that is, significant delocalization of carriers from the core results in trajectories leading far from the origin compared with pseudo-type II regimes that remain close to the origin. Indeed, CdSe/CdS QDs ( Supplementary Fig. 13c,g ), previously shown to allow partial leakage of just the electron into the shell [39] , occupy ROS chart regions between type-II h/e and type-I eh/o regions, whereas CdS/ZnS QDs ( Supplementary Fig. 13b,f ) allow partial leakage of just the hole into the shell and are intermediate between the type-II e/h and type-I o/eh chart regions. Thus, there is theoretically a continuum of possible core–shell combinations of charge carrier localization that can be explored using various material combinations, and this methodology provides rapid analysis of localization of the resulting wavefunctions. 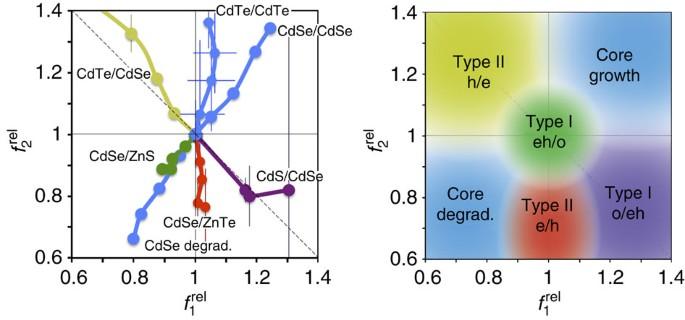Figure 7: Relative oscillator strength phase diagrams showing different localization regimes for charge carriers in core/shell QDs. Left: example experimental data from epitaxial shell growth. Right: summary chart of charge carrier localization regimes from 24 experiments of homoepitaxial shell growth (‘core growth’) and core etching (‘core degradation’) of CdSe and CdTe, as well as shell growth experiments for type-I eh/o materials (CdSe/ZnS, CdSe/CdS, CdS/ZnS), type-I o/eh materials (CdS/CdSe), type-II h/e materials (CdTe/CdSe) and type-II e/h materials (CdSe/ZnTe, CdS/ZnSe). The diagonal dashed line indicates a region for zero net change in combined band edge oscillator strength. Error bars are s.d. Figure 7: Relative oscillator strength phase diagrams showing different localization regimes for charge carriers in core/shell QDs. Left: example experimental data from epitaxial shell growth. Right: summary chart of charge carrier localization regimes from 24 experiments of homoepitaxial shell growth (‘core growth’) and core etching (‘core degradation’) of CdSe and CdTe, as well as shell growth experiments for type-I eh/o materials (CdSe/ZnS, CdSe/CdS, CdS/ZnS), type-I o/eh materials (CdS/CdSe), type-II h/e materials (CdTe/CdSe) and type-II e/h materials (CdSe/ZnTe, CdS/ZnSe). The diagonal dashed line indicates a region for zero net change in combined band edge oscillator strength. Error bars are s.d. Full size image The diagonal dashed line through (1,1) in the ROS chart segregates regions indicative of increasing combined oscillator strength of the first two transitions (towards the top right, ) from those with decreasing combined oscillator strength (towards the bottom left, ). The former generally indicates a decrease in quantum confinement as the exciton spreads over a larger number of atoms, involving more oscillators in the transition (for example, homoepitaxial growth of CdSe/CdSe or CdTe/CdTe). The latter regime indicates a decrease in the number of atoms sharing the wavefunction or a net increase in confinement. Regions along the line simply indicate a redistribution of oscillator strength without a net change in confinement. Importantly, trends in and indicative of different localization regimes become apparent after deposition of just 0.3 monolayers of shell (a fractional monolayer; see Fig. 6e–h ), which is only a small change in nanocrystal structure. Other spectral signatures also become apparent but only after thicker shells are grown. For example, for type II e/h QDs ( Fig. 6d ) the 1st exciton does not substantially shift in energy, and the fluorescence quantum yield is very low (<1%). For type-II h/e QDs ( Fig. 6c ), the 1st exciton peak shifts substantially and the quantum yield can remain high (20% or more). These regimes also exhibit distinct signatures in intraband absorption in the infrared, although such experiments require specialized instruments [40] . It is noteworthy that core–shell materials in which the shell bandgap is smaller than that of the core are problematic to analyse when the shell thickness is greater than approximately one monolayer because of new transitions that arise near the band edge and overlap with the 1st and 2nd exciton peaks. It should be possible to overcome this problem by acquiring spectra at lower temperatures and validating transition energies with PLE spectroscopy. In summary, we have demonstrated that the 1st and 2nd exciton transitions in steady-state absorption spectra of QD heterostructures are sensitive probes for electron and hole localization. Minute changes to electron and hole localization are reflected in alterations in the oscillator strengths of these transitions and can be conveniently visualized on an plot to map the locations of charge carriers during shell growth. When coupled with a simple quantum mechanical model, these spectral signatures can reveal detailed structural changes to the nanocrystal that may not be clearly distinguishable using advanced material characterization techniques, as exemplified for the analysis of Hg x Cd 1−x Te QDs. These methods should improve our understanding of confinement in complex heterostructures that are of considerable current interest derived from cation exchange [30] , [41] , [42] , [43] and seeded growth [44] , [45] , [46] just by monitoring the absorption spectrum. We expect these methods to be widely applicable to four-coordinate direct-bandgap II–VI and III–V materials, and extrapolation to other materials, such as the six-coordinate IV–VI family, should require just an analysis of the 1S–1S transition and any higher order transition with spherical symmetry. Examples here used the most simplistic spherical nanocrystals and wavefunction symmetries; novel properties are expected to arise in structures containing multiple domains with different shapes, such as tetrapod structures in which low energy state are geometrically similar to sp 3 atomic orbitals [47] . This new localization information will be particularly valuable for distinguishing the degree to which the electron and hole are spatially localized in electronic device components to maximize or minimize transfer of particular charge carriers, to maximize or minimize recombination and for determining the degree to which multicomponent structures alloy at their interface. This methodology does not require specialized equipment, and analysis can be easily automated for the observation of incremental structural changes, simply requiring a homogeneous core nanocrystal. These analyses will also be valuable for wavefunction engineering applications to precisely pattern the shapes and spatial locations of charge carrier wavefunctions, and to funnel oscillator strength into specific optical transitions. Core nanocrystal synthesis CdTe QDs were prepared using a high-temperature fast-injection reaction between cadmium tetradecylphosphonate and elemental tellurium in a solvent mixture consisting of oleylamine, trioctylphosphine, diphenylphosphine and octadecene [30] , [48] . By controlling the reaction time, and through the addition of extra precursors, the nanocrystal diameter could be adjusted between 2 and 12 nm with ~10% s.d. in diameter and 25–32 nm full-width-at-half-maximum of the fluorescence emission band. These CdTe nanocrystals were previously found to have zinc blende lattice structures with wurtzite (hexagonal) stacking faults (in 30–40% of the {111} planes) [32] . These nanocrystals showed well-resolved 1st and 2nd exciton peaks (see Fig. 1 and Supplementary Fig. 14 ), and their size-bandgap dependence matched previous correlations as determined through electron microscopy [49] , [50] . Quasi-spherical zinc blende CdS and CdSe nanocrystals were synthesized using methods previously reported in the literature [51] , [52] . Nanocrystals were purified by precipitation from acetone followed by extraction in hexane/methanol. Mercury cation exchange of CdTe→Hg x Cd 1− x Te CdTe nanocrystals were exchanged with mercury using three different methods: organic/fast, organic/slow and aqueous/slow [30] , [48] . Organic/fast: with rapid stirring, a mercury acetate solution in octylamine (0.1 M) was quickly added to a hexane suspension of purified CdTe nanocrystals (20 μM) mixed 1:1 with a solution of oleic acid, oleylamine and hexane (1:1:2 by volume). The solution was monitored via UV–vis absorption spectroscopy until the desired absorption was observed. The nanocrystals were purified by extraction (1:2:3 decane:hexane:methanol). Organic/slow: with rapid stirring, a mercury octanethiolate solution in chloroform (0.1 M) was quickly added to a hexane suspension of purified CdTe nanocrystals (20 μM) containing octylamine (1% by volume). Purification was performed by precipitation from acetone. Aqueous/slow: CdTe nanocrystals were phase-transferred to aqueous solution. A suspension of nanocrystals in chloroform (~20 μM) was mixed with an excess of thioglycerol (~0.2 M) and repeatedly sonicated and vortexed for ~15 min. The nanocrystals were isolated via centrifugation, washed with acetone and then dried under vacuum. After resuspension in a solution of 1 mM thioglycerol in deionized water (pH 11), the nanocrystals were sonicated, centrifuged at 7,000 g for 15 min to remove aggregates and finally passed through a 0.2-μm filter. For mercury exchange, a freshly prepared solution of mercury perchlorate (1 mM) in deionized water was quickly added with rapid stirring to the suspension of nanocrystals (20 μM). Nanocrystals were purified using a centrifugal filtration device (5 kDa molecular weight cutoff). Epitaxial shell growth A purified hexane suspension of nanocrystals (200 nmol) was diluted in a mixture of trioctylphosphine oxide (500 mg, 99%) and octadecene (5 ml). Hexane was removed under vacuum and the mixture was refluxed at 100 °C for 30 min under vacuum and purged with argon. After heating to 160 °C for cadmium-based shells, or 185 °C for zinc-based shells, appropriate precursor solutions (0.1 M) were added dropwise. Precursors were solutions of S (elemental sulfur in octadecene), Se (elemental selenium in octadecene), Te (elemental tellurium with 0.25 M trioctylphosphine in octadecene), Zn (zinc acetate in oleylamine) or Cd (cadmium acetate in oleylamine). Samples were removed with a needle, diluted in chloroform and purified by acetone precipitations before characterization. Instrumentation Absorption spectra were measured using a Shimadzu UV-2401PC scanning spectrophotometer (300–900 nm) or an Ocean Optics NIR-512 spectrometer with tungsten halogen lamp (850–1,700 nm). Room-temperature steady-state fluorescence spectra were obtained at using a Photon Technology International spectrofluorometer with photomultiplier tube for the 400–800 nm spectral range and InGaAs detector for 800–1,700 nm. Photoluminescence excitation spectroscopy was performed using a Horiba Nanolog UV–vis-NIR spectrofluorometer (240–1,550 nm) with internal excitation intensity correction and photomultiplier tube for the 400- to 800-nm spectral range and InGaAs detector for 800–1,550 nm. PLE spectra were obtained at 0 °C using a cell immersed in an ice water bath. Room-temperature Raman spectra were obtained using a Spex Triplemate microscope with Princeton Instruments CCD detector and 532-nm laser excitation. Samples were cast from hexane solutions on aluminum slides. For X-ray diffraction, dried solid nanocrystals from hexane solutions were analysed using a PANalytical X-Pert PRO with Cu X-ray source. For electron microscopy and EDX spectroscopy, samples were prepared from a hexane suspension of purified nanocrystals (5 μl) dropped on formvar/carbon 200 mesh TEM grids. Normal resolution TEM imaging was performed with a Hitachi H-7500 TEM. High-resolution images were obtained using a Tecnai F30 with Oxford EDX 6763 attachment (in the lab of ZL Wang, supported by NSF funding DMR 0922776). For elemental analysis, purified aqueous nanocrystals were dissolved with the addition of a small amount of nitric acid; hydrophobic nanocrystals in nonpolar solvents were purified with acetone precipitations, dried under vacuum, dissolved in aqua regia at 80 °C for ~4 h and diluted in deionized water. Solutions were analysed for cadmium, mercury and tellurium using ICP-MS (VG PlasmaQuad 3). Elemental analysis To simplify studies of Hg x Cd 1− x Te nanocrystals without the need to characterize all samples for composition, we performed ICP-MS analysis on six different CdTe sizes (2.3, 3.0, 4.0, 4.9, 6.1 and 8.4 nm) before and after mercury cation exchange to establish spectral relationships. The aqueous exchange procedure allowed for efficient purification from excess mercury for ICP-MS. The fraction of mercury ( x ) incorporated into the nanocrystals scaled nearly linearly with the absorption cross-section at high energy for all six nanocrystal sizes subjected to cation exchange in water. The value of x could be calculated using the following equation: where A CdTe is the absorption of the CdTe QDs at 4.0 eV and A alloy is the absorption after mercury exchange, assuming that the QD concentration does not change and that the same number of atoms are in the CdTe nanocrystals as are in the resulting Hg x Cd 1− x Te nanocrystals. Empirical oscillator strength determination For the analysis of CdTe QDs, we calculated absolute oscillator strengths by first acquiring absolute absorption coefficient spectra. Absorption spectra were obtained for suspensions of nanocrystals with experimentally measured concentration and diameter. Spectra were then plotted as absorption coefficient ( α , cm − 1 ) versus frequency ( ν , s − 1 ), validated through convergence with the spectrum of bulk CdTe (corrected for local field effects) at high energy where energy bands are nearly continuous (3.3–4.0 eV) because quantum confinement effects are small ( Supplementary Fig. 14 ) [33] , [50] , [53] . Each spectrum was then fit to a sum of Gaussian functions using the method of Klimov [33] : where there are a total of n Gaussian functions (that is, transitions), i , each with an area of a i (cm − 1 s − 1 ) and centroid frequency ν i (s − 1 ). d R is the relative s.d. of the nanocrystal radius and ν g (s − 1 ) is the bandgap frequency of the bulk material. Best fits of a i , ν i and d R were calculated using the least squares method. Initial guesses for ν i values were determined from the minima of the 2nd derivative of the spectrum or maxima of the 4th derivative of the spectrum (see detailed description in Supplementary Methods and Supplementary Figs 15–21 ). Values of a i and d R were unbounded, but ν i was typically bound to ±50 meV of the initial guess. All calculations were performed using an automated Matlab script. The values of a i were converted to absolute oscillator strengths ( f 1 ) with the following formula [54] : where m e is the electron mass, ε o is the permittivity of free space, c is the speed of light, e is the elementary charge, h is the Planck constant and r is the nanocrystal radius. To determine f rel values, absorption spectra were simply obtained from equal-concentration QD solutions. In this case, absorption spectra were not normalized to absorption coefficient, yielding an effective value of each transition peak a i . Thus, and for the core. EMA Nanocrystals were modelled using the EMA and assumed to be spherically symmetric and with finite energy wells. Nanocrystals were modelled with N total concentric layers ( L ), with increasing L value from the core ( L =1) to the surroundings ( L = N ), with discrete boundaries between layers. Radial distances for each layer were designated as r L , with material parameters for each layer specified in Supplementary Table 1 . For non-interacting models of s-type wavefunctions ( l =0) of the electron and hole, we use the method of Haus et al. [24] , with Coulombic terms included as perturbations included for bandgap calculations, ignoring interfacial polarization terms that were found to be small. Calculations begin with the time-independent Schrödinger equation in three dimensions: where E K is the kinetic energy of the electron or hole, E P is its potential energy, m is its mass and ħ is the reduced Planck constant. The radial and angular components of the wavefunction are separated: where for ℓ = m ℓ =0 and R ( r ) has solutions of the form [24] Here j ℓ ( k L r ) is a spherical Bessel function, n ℓ ( k L r ) is a spherical Neumann function and k L is the wavevector of the electron or hole in layer L , defined by the equation where E P, L is its potential energy and m L is its mass in layer L. We use the boundary conditions that is continuous at all layer interfaces, and is continuous at all layer interfaces, modulated by changes in effective mass. Thus, B 1 =0 and R ( r N )=0. This results in a system of 2 N −1 linear equations with coefficients A L and B L for each layer L (2 N −1 unknowns), allowing solution for E K of each carrier, E K,e and E K,h , as well as the wavefunctions and , which must be normalized according to: where d τ =d x d y d z . To determine the bandgap we account for Coulombic interactions between the electron and hole as a perturbation [55] : where e is the elementary charge, ε is the dielectric constant, is the vector position of the electron and is the vector position of the hole. Thus, the bandgap is E g,nanocrystal = E g,bulk + E K,e + E K,h + E c . Noninteracting wavefunction overlap, φ , was calculated as: Oscillator strength calculations with interactions The wavefunctions of the 1S(e)1S(h) and the 1S(e)2S(h) transitions of the alloyed and core–shell particles were calculated through the variational principle using the Rayleigh ratio. First, the wavefunctions of the non-interacting electron, , and hole, , were separately solved numerically via a Verner’s 8–9th order Runge Kutta scheme according to the potential profile cases described above. By superposition, these solutions were combined with a Coulombic interaction expression using a form similar to previous microcrystal calculations performed by Kayanuma [56] , where α is the variational parameter. This leads to the complete transition wavefunction of the form The variational parameter for each transition wavefunction is solved by numerical integration to find the interaction energy as a function of α , then finding the value of α where the interaction energy is at a minimum. Once the transition wavefunction is known, by considering the approximation of the oscillator strength of the exciton derived by Henry and Nassau [57] one obtains the proportionality Thus, ratios of the oscillator strength of a Hg x Cd 1− x Te particle after cation exchange ( f ) to a pure CdTe particle ( f 0 ) were calculated where, for a core/shell example, the 1S(e)2S(h) transition is represented by For both models we have focused on the heavy holes; light holes are also expected to contribute, although to a much smaller extent [58] ; a model incorporating multiple hole states will likely further improve accuracy. It is also important to note the poor accuracy of the EMA for small particles under strong confinement because of non-parabolic shapes of the energy band dispersion curves at high energy. In order to model homogeneously alloyed Hg x Cd 1− x Te nanocrystals the well depth and material properties were simply determined using Vegard’s Law. For core–shell CdTe/HgTe nanocrystals, we must account for fractional monolayers for small quantities of mercury incorporated. It is thus assumed that a single monolayer will develop first following Vegard’s law for this outer well. Then, once mercury has completely replaced the cadmium in the first monolayer, a second monolayer adjacent to the first monolayer nearer to the core will begin to develop in the same manner. How to cite this article: Smith, A. M. et al. Mapping the spatial distribution of charge carriers in quantum-confined heterostructures. Nat. Commun. 5:4506 doi: 10.1038/ncomms5506 (2014).